Flammable biomes dominated by eucalypts originated at the Cretaceous–Palaeogene boundary Fire is a major modifier of communities, but the evolutionary origins of its prevalent role in shaping current biomes are uncertain. Australia is among the most fire-prone continents, with most of the landmass occupied by the fire-dependent sclerophyll and savanna biomes. In contrast to biomes with similar climates in other continents, Australia has a tree flora dominated by a single genus, Eucalyptus , and related Myrtaceae. A unique mechanism in Myrtaceae for enduring and recovering from fire damage likely resulted in this dominance. Here, we find a conserved phylogenetic relationship between post-fire resprouting (epicormic) anatomy and biome evolution, dating from 60 to 62 Ma, in the earliest Palaeogene. Thus, fire-dependent communities likely existed 50 million years earlier than previously thought. We predict that epicormic resprouting could make eucalypt forests and woodlands an excellent long-term carbon bank for reducing atmospheric CO 2 compared with biomes with similar fire regimes in other continents. Open-canopied communities are far more extensive across the world than predicted by consideration of climate and soil fertility alone [1] . Moreover, boundaries between open woodlands and closed-canopy rainforest are often surprisingly sharp [1] , [2] . Fire is known to have a major role in maintaining open communities: both plot experiments and modelling show that, in the absence of fire, closed forests would cover much of both Australia [2] , [3] and the world [1] —hence their definition as 'fire-dependent' [1] . In Australia this effect is extreme, with rainforest marginalized by fire to a tiny portion (2%) of the continent and absent from much of the climatically and edaphically suitable landscape [2] . Even the vast central Australian arid zone is dominated by fire [4] , [5] at frequencies similar to those in temperate grassy woodlands and dry sclerophyll forests [6] (global modelling suggesting that this region is 'bare' [1] is simplistic). In contrast with other continents, a single diverse family, Myrtaceae, dominates Australian fire-dependent woodlands and forests, with 1,600 species, including 800 eucalypts and their close relatives [7] . Many are excellent post-fire epicormic resprouters from the stems and branches after high-intensity fires [8] , [9] , [10] , [11] . In most investigated angiosperm trees, dormant epicormic buds are situated in the outer bark [8] , [12] , where they are likely killed by fire, but in eucalypts, the epicormic bud-forming structures are located deeply, where they are protected by the full thickness of the bark and can sprout even after high-intensity fires [8] . Moreover, the epicormic structures of eucalypts appear unique, consisting not of buds but of narrow, radially oriented strips of cells of meristematic appearance, and as such differ from those recorded in other families [8] , [9] , [10] , [11] . Given the above, it has been hypothesized that evolution of fire tolerance in Myrtaceae was directly linked with the origins and expansion of the fire-dependent biomes in Australia, especially the southern sclerophyll and northern savanna biomes [2] , [6] , [13] . However, the influence of wildfire on the evolution of Australian biomes through the Palaeogene, when Australia was still part of East Gondwana, has been little studied. The Australian fossil record has provided little direct evidence of fire (fusain charcoal) before the mid-Miocene, when the climate aridified and charcoal levels increased dramatically [2] , [14] . Here, we show that specialized epicormic resprouting originated in the eucalypt lineage much earlier, at least 60 million years ago. We find a significant link between the evolution of this unique anatomy and the timing of shifts by Myrtaceae into the flammable sclerophyll biome. However, there was no statistical association with the more recent shifts into the monsoonal biome, which experiences more frequent but less intense fires. Our results contrast with the current view that fire-dominated vegetation originated much later, after global climate aridified and the monsoonal biome developed, in the late Miocene [14] , [15] , [16] . 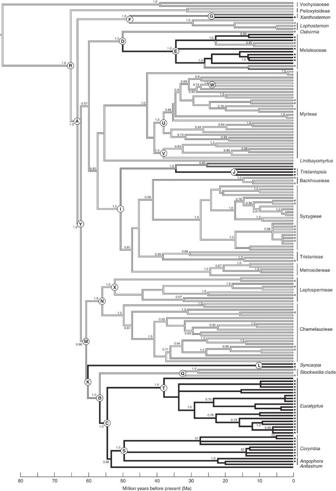Figure 1: Inferred evolutionary history of post-fire epicormic resprouting mapped onto a Bayesian phylogeny of Myrtaceae. Time scale is millions of years before present (Ma). Labels indicate higher taxa mentioned in the text. Shading of boxes at tips indicates scoring for the trait 'likely epicormic resprouter' (black), 'likely non-resprouter' (white) or not scored (no box). Ancestral states reconstructed by parsimony are shown at internal branches; grey indicates an equivocal reconstruction. Nodes labelled with upper case letters in circles are for reference from the text and tables. Decimal values on branches indicate Bayesian posterior probabilities; integers (inCorymbia) indicate parsimony bootstrap scores. Ancestral biomes and epicormic structures Using trait mapping on a dated molecular phylogeny, we found that both epicormic resprouting in Myrtaceae and their adaptation to the sclerophyll biome probably evolved in the earliest Palaeogene, 60–62 Ma ( Figs 1 and 2 ; Table 1 ; Supplementary Figs S1 and S2 ). The myrtoid ancestor reconstructs as a non-resprouting inhabitant of rainforest ( Table 1 ; Fig. 1 ; Supplementary Fig. S2 ). Thus, fire-dependent sclerophyll communities likely existed 50 million years before the well-documented late-Miocene expansion of fire-dependent biomes [14] , [15] , [16] . We tested the hypothesis that protection of epicormic regenerative tissue in Myrtaceae is positively correlated with flammability of habitat. Using phylogenetically independent contrasts, we found that these traits are correlated (Pagel94 maximum likelihood (ML) test, P =0.027; Bayesian stochastic mapping test, P <0.000001). Figure 1: Inferred evolutionary history of post-fire epicormic resprouting mapped onto a Bayesian phylogeny of Myrtaceae. Time scale is millions of years before present (Ma). Labels indicate higher taxa mentioned in the text. Shading of boxes at tips indicates scoring for the trait 'likely epicormic resprouter' (black), 'likely non-resprouter' (white) or not scored (no box). Ancestral states reconstructed by parsimony are shown at internal branches; grey indicates an equivocal reconstruction. Nodes labelled with upper case letters in circles are for reference from the text and tables. Decimal values on branches indicate Bayesian posterior probabilities; integers (in Corymbia ) indicate parsimony bootstrap scores. 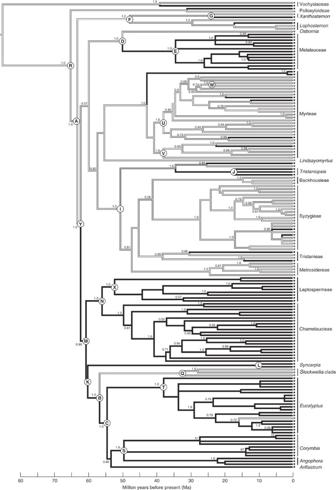Figure 2: Inferred evolutionary history of biome flammability mapped onto a Bayesian phylogeny of Myrtaceae. Time scale is millions of years before present (Ma). Labels indicate higher taxa mentioned in the text. Shading of boxes at tips and along branches indicates scoring for the trait 'biome flammable' (black) or 'non-flammable' (white). Ancestral states reconstructed by parsimony are shown at internal branches; grey indicates an equivocal reconstruction. Nodes labelled with upper case letters in circles are for reference from the text and tables. Decimal values on branches indicate Bayesian posterior probabilities; integers (inCorymbia) indicate parsimony bootstrap scores. Full size image Figure 2: Inferred evolutionary history of biome flammability mapped onto a Bayesian phylogeny of Myrtaceae. Time scale is millions of years before present (Ma). Labels indicate higher taxa mentioned in the text. Shading of boxes at tips and along branches indicates scoring for the trait 'biome flammable' (black) or 'non-flammable' (white). Ancestral states reconstructed by parsimony are shown at internal branches; grey indicates an equivocal reconstruction. Nodes labelled with upper case letters in circles are for reference from the text and tables. Decimal values on branches indicate Bayesian posterior probabilities; integers (in Corymbia ) indicate parsimony bootstrap scores. Full size image Table 1 Estimated timing of transitions in epicormic and biome traits. Full size table Biome transitions We tested whether the variables in question are phylogenetically conserved, because biome conservation has been demonstrated previously in eucalypts [17] , and conservation of post-fire persistence traits has been found in taxa occurring in fire-dependent communities. Biome adaptations in the Myrtaceae are significantly conserved (tip randomization test, P <0.001) and the transitions that have occurred are strongly directional—all sclerophyll lineages originated from a rainforest ancestor and all monsoonal savanna lineages arose more recently, from sclerophyll or rainforest ancestors. Two-thirds (21) of biome shifts were into savanna, confirming that this biome is a sink relative to the other biomes and suggesting that the advent of monsoonal climate opened a major ecological opportunity that pre-adapted Myrtaceae were able to exploit effectively. However, we found no support for the hypothesis that this new environment (with its more frequent but less intense fires [6] , [18] ) exerted sufficient selection to alter the epicormic anatomy of the Myrtaceae overall (Pagel94 ML test, P =0.137; Bayesian stochastic mapping test, P =0.2), except in Xanthostemon and perhaps Melaleuca ( Supplementary Fig. S1 ). By contrast, five of the seven transitions in epicormic resprouting anatomy coincided with shifts between the everwet and sclerophyll biomes ( Table 1 ). Alternative reconstructions The sequence of events at the base of the eucalypts is unclear because of uncertain trait reconstructions at nodes M and K ( Figs 1 and 2 ; Supplementary Figs S1 and S2 ) and lack of support for the position of Syncarpia . The inferred trait transitions shown in Table 1 are a shift into the sclerophyll biome with a gain of resprouting epicormic type A between nodes Y and K, and a reversal of both traits in the Stockwellia clade (node Q). The alternative reconstruction infers an independent transition to sclerophyll and epicormic resprouting in each of Syncarpia and Eucalypteae, with retention of the ancestral everwet biome and epicormic resprouting in the Stockwellia clade. The timing of these alternative reconstructions (62–55 Ma) is about the same as in the reconstructions shown in the Figures and Table 1 . The lack of branch length data for interpolated species within Syncarpia , Tristaniopsis and Xanthostemon resulted in wide bounds on the timing estimates of transitions within these lineages ( Table 1 ). Reversals to non-resprouting types occurred within Melaleuca , whose most recent common ancestor reconstructs as a resprouter occurring in the sclerophyll biome. The timing of these shifts is uncertain because of lack of branch length information within the group. We have shown that both epicormic resprouting in Myrtaceae and flammable sclerophyll biomes likely originated in the earliest Cenozoic, 60–62 Ma, and that their evolution is significantly linked. In eucalypts, the distinctive epicormic resprouting anatomy has been strictly conserved until the present, despite changes in habitat and response to fire. For example, Eucalyptus brachyandra grows on fire-protected cliffs and E. regnans dominates wet sclerophyll forest and, although usually killed by high-intensity fires, still retains capacity to resprout epicormically after less intense fires [10] . Sclerophyllous morphology is often assumed to be an adaptation to fire and a driver of diversification [13] , [19] , [20] , but sclerophylly has diverse functions and is not necessarily an indicator of climates in general or fire-prone vegetation in particular [2] , [21] , [22] . Nevertheless, in Australia, the unique epicormic anatomy (types A and B: Supplementary Table S1 ) of Myrtaceae, especially eucalypts, is known to be responsible for post-fire recovery [8] , [9] , [11] . Although scleromorphy in the Australian flora dates back to the late Cretaceous [21] , there is little direct charcoal fossil evidence for wildfire until the late Miocene [14] . Hence, it has been widely assumed that fire-dominated biomes became extensive only when the global climate aridified and became more seasonal after 15 Ma [1] , [2] , [14] . In other parts of the world, there is charcoal evidence that, in the lead-up to the Palaeocene–Eocene thermal maximum at 55 Ma, fire frequency increased [23] , with global atmospheric oxygen levels above those of the present [24] . During this period, seasonally hot and dry climates originated both in Australia [25] and elsewhere [26] , and such climates are characterized by fires ignited by electrical storms [2] . Our results suggest, independently of the fossil record, that fire-dominated communities were present in Australia during this period. Limited palaeontological evidence suggests that a monsoonal climate might have originated in Australia by 30 Ma [18] , [27] . Some of the shifts into savanna inferred for Myrtaceae could have occurred before 30 Ma, in the Oligocene or Eocene ( Supplementary Fig. S2 ); however, all monsoonal lineages have long stems that terminate in the Miocene or even in the present. As a transition could have occurred at any point along a lineage stem, none positively indicates a pre-Miocene origin of savanna ( Supplementary Fig. S2 ). Multiple lines of evidence show that the savanna biome expanded worldwide in the late Miocene [15] , [16] and our results for Myrtaceae are consistent with this. Did the Myrtaceae make the flammable biomes or vice versa ? These two alternatives make different predictions. If fire drove evolutionary change, one might expect multiple consequent origins of the trait that conveys tolerance. Alternatively, if the dominance of Myrtaceae led to biome flammability, this could have resulted from a single preceding shift to epicormic resprouting in the family. Foliar glands that produce aromatic oils are found throughout Myrtaceae, and probably evolved in their ancestor as a toxic defence against herbivores and also promoted flammability of plants [28] . Thus, epicormic resprouting could be the result of selection originating as a by-product of a defense system. However, our data show multiple origins of resprouting in Myrtaceae: once in each of Melaleuca , Tristaniopsis and Xanthostemon and once or twice in the eucalypt– Syncarpia lineage ( Fig. 1 ), favouring the hypothesis that flammable biomes originated first. There is no evidence that the epicormic change preceded the shift to a flammable biome in any lineage; rather, the biome transition apparently occurred before the epicormic change in the eucalypt– Syncarpia lineage (see, Supplementary Figs S1 and S2 ). A third possibility combines these scenarios. Myrtaceae could have risen to dominance first, favouring a fire regime that then selected for epicormic shifts in multiple lineages, thus initiating a feedback loop that maintained or increased the dominance of Myrtaceae. The eucalypts appear to be the key to the rise to dominance of the Myrtaceae in Australia. Why then have eucalypts not taken over the seasonally dry regions of the world? During the Miocene, eucalypts were present in New Zealand and Southeast Asia in association with other sclerophyll and xeric flora, such as acacias, chenopods and Casuarinaceae [7] , [29] , [30] . At this time, there was an abundance of charcoal, indicating frequent burning in these communities [29] , [30] . Multiple crown-group eucalypt lineages were also present in Patagonia during the early Eocene [31] . They persist in Southeast Asia today, but have since gone extinct in New Zealand and Patagonia, likely as a result of climate change to wetter and colder conditions that are no longer so prone to fire [19] , [32] . Dispersal limitation may account for the lack of spread of eucalypts beyond the immediate region since the end of the Eocene, when Australia separated from East Gondwana. Recently, it was suggested that eucalypts could make a large contribution to carbon sequestration in a future greenhouse world, based on a demonstrated positive growth response to an elevation of either atmospheric CO 2 or temperature [33] . Our results independently predict that eucalypt forests and woodlands could be a superior long-term carbon bank compared with climatically similar fire-dependent biomes in other continents. By resprouting from the trunk and branches, eucalypts preserve most of their aboveground woody biomass after wildfires, both in northern savanna [3] and in sclerophyll forest of the temperate southeast [34] . In contrast, other trees that do not resprout epicormically lose their aerial wood after high-intensity fire (as opposed to lower-intensity fires, which their stems might survive). Consequently, in non-epicormic resprouters, the woody biomass decays and the stored carbon is released after the fire. Such trees either resprout from the base or are killed and regenerate from seed [35] , [36] . They recover more slowly than eucalypts after fire [37] and are forced to accumulate aboveground wood from scratch. When a pine forest planted for carbon capture burns, the trees die and the carbon bank drains. Phylogenetics A dated molecular phylogeny of Myrtaceae was constructed using 66 species with known epicormic anatomy ( Supplementary Table S1 ) and 97 additional taxa, totalling 163 terminals representing higher taxa across the family, on the basis of a recent phylogenetic classification of the family [38] . Most deep-level phylogenetic diversity in the family is found within Australia (for example, 14 of 15 tribes in subfamily Myrtoideae), but we also sampled extra-Australian members of these (where applicable) and the sixteenth tribe (Metrosidereae) to ensure representation of their geography and biomes. Additionally, we sampled both genera of subfamily Psiloxyloideae and of the sister group, Vochysiaceae. The phylogeny was constructed in two stages. First, sequences of 111 taxa of ITS (internal transcribed spacers of nuclear ribosomal DNA), matK and ndhF from Genbank ( Supplementary Table S3 ) were aligned and concatenated after checking for pseudogenes (ITS) and conflicts between data partitions. A rate-smoothed phylogeny, in which branch lengths were proportional to time (chronogram), was derived using Bayesian inference in BEAST [39] , ver. 1.5.4. The alignment was divided into seven partitions: ITS, 5′ flanking region of matK , first codon sites of matK , second codon sites of matK , third codon sites of matK , first codon sites of ndhF , second codon sites of ndhF and third codon sites of ndhF . Each partition was assigned an independent General Time Reversible model of nucleotide substitution, chosen using the Bayesian information criterion, as calculated using Modelgenerator [40] . Rate variation among lineages was modelled using an uncorrelated lognormal relaxed clock and a birth–death process was used for the tree prior probability distribution. Posterior distributions of all parameter values, including the tree, were estimated via Markov chain Monte Carlo (MCMC) sampling. Three replicate MCMC runs were performed, with the tree and parameter values sampled every 5×10 3 steps over a total of 5×10 7 steps. Tracer 1.5 (ref. 41 ) was used to assess convergence between runs and to estimate an appropriate number of samples to discard as burn-in by ensuring that effective sample sizes were sufficient (that is, >200) to provide reasonable estimates of model parameter variance. This was done by progressively discarding samples until all effective sample sizes exceeded 200. Posterior samples from the three independent runs were combined and the trees and parameter values were summarized. The sampled tree with the maximum product of clade credibilities was identified using TreeAnnotator [39] and viewed using FigTree 1.3.1 (ref. 42 ). The phylogeny was estimated both with and without internal constraints to test whether calibration affected the topology [43] . Calibration of the relaxed molecular clock To estimate absolute divergence times, the analysis was calibrated using pollen fossils of known age placed at seven internal nodes. Fossil pollens suitable for calibration were identified using a backbone-constraint test [19] . This method searches for the most parsimonious placement of fossil pollens on a molecular phylogeny, using a pollen character data matrix scored for the terminal taxa. A total of 26 pollen fossils were added one at a time to a morphological matrix containing 111 extant taxa and 11 pollen characters. The phylogenetic placement of each fossil on the unconstrained molecular phylogeny was estimated using heuristic parsimony searches of 100 random-addition replicates with tree-bisection-reconnection in PAUP* [44] , with the tree-search constrained by the molecular phylogeny estimated without internal calibrations. As suggested [19] , the most parsimonious +1 and +2 trees were also saved, to assess confidence of fossil placements. The test identified seven fossils as suitable for calibration ( Supplementary Table S2 ). In cases in which more than one fossil was placed at a given node, the oldest was used for calibration. Nodes used as calibration points ( Supplementary Table S2 ) were constrained to be monophyletic in the BEAST analysis; all these nodes were supported in the unconstrained analysis. A prior distribution (lognormal or normal) was assigned to each calibration point, as recommended [43] . The root of the tree, being the stem node of Myrtaceae, was calibrated with a normally distributed age estimate of 85 Ma with s.d.=2.5 ( Supplementary Table S2 ). We used the fossil Myrtaceidites mesonesus (61 Ma) to calibrate the crown of Myrtaceae instead of M. lisamae ( ∼ 86 Ma), used previously [45] , because the backbone-constraint test [19] indicated that the latter was probably misplaced as a member of the Myrtaceae crown. Recently, 52-Ma Eucalyptus macrofossils were discovered in Patagonia [31] and are older than our 37 Ma constraint ( M. eucalyptoides , Supplementary Table S2 ) for the crown node of the genus. However, we could not use the Patagonian fossils as a constraint because morphological descriptions needed to place them on the phylogeny are not yet published. If we had been able to use these fossils as a constraint, our dating estimates could have been even older, implying even earlier origins of flammability. Interpolation of taxa with known anatomy In the second stage of the phylogenetics, 52 taxa with known epicormic anatomy ( Supplementary Table S1 ), but lacking sequence data, were interpolated by hand into the chronogram ( Figs 1 and 2 ; Supplementary Figs S1 and S2 ) on the basis of their position in other phylogenies, that is, eucalypts [27] , [46] , [47] , Melaleuca [48] , Syzygium s.l . [49] and Myrtaceae, using matK only [38] . Chronological branch lengths were unavailable for some interpolated taxa and, in these cases, branch lengths were arbitrarily equalized above and below the interpolated nodes. This did not affect the inferences of trait evolution in the eucalypt lineage because the transitions to flammability occurred near the base of the tree, where branch length information was available. However, branch length uncertainty within Syncarpia , Tristaniopsis and Xanthostemon resulted in wide bounds on the timing estimates of transitions within these lineages ( Table 1 ). Epicormic anatomy We scored a matrix for five epicormic structural types across 66 myrtaceous taxa studied to date [8] , [9] , [10] , [11] , [50] and for their biome of occurrence ( Supplementary Table S1 ). In the first (type A), the bud-forming cells comprise meristem strips (that is, radially oriented strips of cells of meristematic appearance) and are present at all depths in the bark, and in most cases probably extend a short distance into the outer secondary xylem. For the available bark thickness, this structure provides the maximum heat protection for the bud-forming cells. In the second type (B), the epicormic buds or bud-forming meristems are located close to the cambial surface and covered by numerous layers of dead bark (paperbarks). The papery structure provides maximum heat protection for the bud-forming cells, but buds need to emerge through numerous bark layers. In the third type (C), epicormic buds are located at the base of a narrow depression in the bark and are thus about halfway between the bark surface and the cambial surface. This provides an intermediate level of protection for the available bark thickness. In the fourth type (D), epicormic buds are situated at or near the bark surface, giving minimal protection from the heat of a fire. In the fifth type (E), epicormic bud-forming structures are apparently absent. Various processes have been implicated in the death of epicormic buds or failure in their initial development [10] . Trait evolution These data were imported into Mesquite ver. 2.7 (ref. 51 ) and SIMMAP ver. 1.5 (ref. 52 ) together with the phylogeny constructed as above. Some of the statistical tests used in Mesquite required binary variables; hence, the epicormic character was rescored to indicate whether the anatomy of each species indicated a likely (types A–C) or unlikely (types D and E) epicormic resprouter after a moderate-to-intense fire, on the basis of the degree of protection given to the epicormic buds and meristems ( Supplementary Table S1 ). Similarly, the biomes were rescored according to whether they are fire-dependent (subject to recurrent fires, that is, monsoonal savanna and southern sclerophyll) or not (everwet, that is, rainforest and mangrove). Additionally, all 163 taxa in the phylogeny were scored for the biome and flammability characters, whether their epicormic traits were known or not. Ancestral states of each trait were reconstructed at the crown node of Myrtoideae, as well as the number and timing of transitions in each trait, using the parsimony and ML models in Mesquite. In Mesquite, likelihood ratio tests determined that the single transition-rate model, Mk1 [53] , sufficed for the epicormic traits, whereas the Mk2 model (with differential forward and reverse rates) was a significantly better fit for the biome traits. Comparative hypothesis tests A primary aim of this study was to test whether protection of epicormic regenerative tissue in Myrtaceae is positively correlated with flammability of habitat. First, we tested whether the variables in question are phylogenetically conserved, because biome conservation has been demonstrated previously in eucalypts [17] and conservation of post-fire persistence traits has been found in taxa occurring in fire-dependent communities [54] . Phylogenetic conservatism of all four traits was tested in Mesquite using a null distribution generated from 1,000 randomizations of the tips of the phylogeny, with parsimony tree length as the test variable [17] . Significant results ( P <0.001) from all these tests indicated that a tree-based correlation test was necessary to assess the relationship between the traits. We used the Pagel94 implementation in Mesquite of Pagel's [55] test, which takes phylogenetic conservatism into account. As recommended, we generated a null distribution using 1,000 simulations and set the number of iterations of the likelihood estimation to 20, rather than the default 8. For testing the primary hypothesis, the Y (dependent) variable was 'likely resprouter/not' and the X (independent) variable was 'biome fire-dependent/not'. The same test was used to address the question whether taxa in the monsoonal savanna biome are less likely to have resprouting epicormic anatomy than those in the southern sclerophyll biome, that is Y ='likely resprouter/not' and X ='biome savanna/sclerophyll'. In this case, taxa occurring in rainforest were irrelevant and eliminated from the analysis. These tests were repeated using Bayesian stochastic mapping as implemented in SIMMAP ver. 1.5 (ref. 52 ). The advantage of the Bayesian approach over parsimony and ML mapping is that uncertainty in parameters can be accommodated by using MCMC samples from their respective posterior distributions [56] . We accepted default prior values for the transition bias (β, uninformative, α =1.0), γ and MCMC sampling parameters. How to cite this article: Crisp, M. D. et al . Flammable biomes dominated by eucalypts originated at the Cretaceous–Palaeogene boundary. Nat. Commun. 2:193 doi: 10.1038/ncomms1191 (2011).